Evolution of Landau levels into edge states in graphene Two-dimensional electron systems in the presence of a magnetic field support topologically ordered states, in which the coexistence of an insulating bulk with conducting one-dimensional chiral edge states gives rise to the quantum Hall effect. For systems confined by sharp boundaries, theory predicts a unique edge-bulk correspondence, which is central to proposals of quantum Hall-based topological qubits. However, in conventional semiconductor-based two-dimensional electron systems, these elegant concepts are difficult to realize, because edge-state reconstruction due to soft boundaries destroys the edge-bulk correspondence. Here we use scanning tunnelling microscopy and spectroscopy to follow the spatial evolution of electronic (Landau) levels towards an edge of graphene supported above a graphite substrate. We observe no edge-state reconstruction, in agreement with calculations based on an atomically sharp boundary. Our results single out graphene as a system where the edge structure can be controlled and the edge-bulk correspondence is preserved. The gapless one-dimensional chiral edge states near the boundaries of a two-dimensional (2D) electron system (2DES) in the quantum Hall (QH) regime host chiral charge carriers, where the right- and left-moving species reside on opposite edges [1] , [2] , [3] . As a result, backscattering is suppressed for well-separated edges [4] , leading to robust one-dimensional ballistic channels that provide an ideal laboratory for quantum transport in one dimension [5] , [6] , [7] . In particular, the edge states of topologically ordered 2DES exhibiting the QH effect are expected to display an edge-bulk correspondence, which is currently much sought after because of its pivotal role in QH-based quantum computing [8] , [9] , [10] . However, in the semiconductor-based 2DES studied thus far, this ‘topologically protected’ correspondence is notoriously difficult to realize [11] , [12] . The most likely cause of the discrepancy between theory and experiment is the generic occurrence of edge reconstruction [13] , [14] , [15] , [16] , [17] , [18] , [19] , [20] , [21] , [22] , [23] in the semiconductor 2DES, which induces additional edge modes that are not tied to the bulk topology and disrupt the predicted universality [24] . In these systems, the lithographically defined edges have soft confinement potentials, caused by the gates and dopant layer being far away from the 2DES, which favour the reconstruction of the edge states into alternating compressible and incompressible strips ( Fig. 1a ). This obscures the universal behaviour expected for edge states [18] and is problematic for applications, which rely on the topological properties of the edges [8] , [9] , [10] . 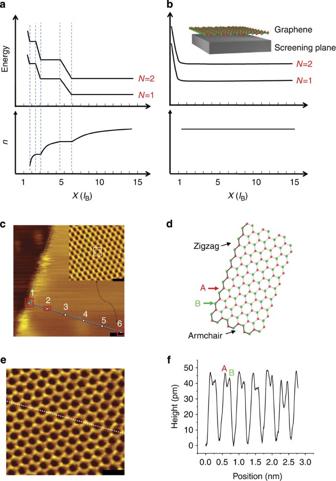Figure 1: Edges and LLs and graphene structure. (a) Edge reconstruction in semiconductor-based 2DES. The distances from gates and screening plane are much larger than the magnetic length. Top: spatial variation of LL energy as a function of distance from the edge shows the effect of edge-state reconstruction. Dashed lines mark the boundary between compressible and incompressible strips. Bottom: spatial variation of the reconstructed carrier density close to the edge. (b) Same as inafor graphene and distances from screening planes that are much smaller than the magnetic length. Inset: schematic illustration of graphene sample and screening plane. (c) STM of a graphene flake on a graphite substrate near a zigzag edge measured in a field of 4 T at 4.4 K. Inset: the edge type is determined from atomic-resolution STM at a distance of ~32 nm=2.5lBfrom the edge (position 6 ). The dashed line marks a zigzag direction and is parallel to the edge, also marked with a dashed line in the main panel. LL spectra taken at intervals of 0.5lB(at the positions marked 1–6) and averaged over an area 0.4 × 0.4 nm2(marked by the white square in the inset for position 6) are shown inFig. 2. Scale bars: 5 nm (main panel), 500 pm (inset). The rectangles at position 1, 2 and 6 indicate the areas of the topography maps inFig. 4and the inset. (d) Graphene edges. The two sublattices in the honeycomb structure are denotedAandB. The zigzag edge termination contains eitherA- orB-type atoms, whereas the armchair contains both types. (e) Atomic-resolution STM topography measured far from the edge shows the honeycomb structure with a slight intensity asymmetry on the two sublattices. Scale bar: 500 pm. (f) Intensity plot taken along the line in paneledisplays an intensity modulation where one of the sublattices, markedA, appears 10% less intense than the other markedB. Figure 1: Edges and LLs and graphene structure. ( a ) Edge reconstruction in semiconductor-based 2DES. The distances from gates and screening plane are much larger than the magnetic length. Top: spatial variation of LL energy as a function of distance from the edge shows the effect of edge-state reconstruction. Dashed lines mark the boundary between compressible and incompressible strips. Bottom: spatial variation of the reconstructed carrier density close to the edge. ( b ) Same as in a for graphene and distances from screening planes that are much smaller than the magnetic length. Inset: schematic illustration of graphene sample and screening plane. ( c ) STM of a graphene flake on a graphite substrate near a zigzag edge measured in a field of 4 T at 4.4 K. Inset: the edge type is determined from atomic-resolution STM at a distance of ~32 nm=2.5 l B from the edge (position 6 ). The dashed line marks a zigzag direction and is parallel to the edge, also marked with a dashed line in the main panel. LL spectra taken at intervals of 0.5 l B (at the positions marked 1–6) and averaged over an area 0.4 × 0.4 nm 2 (marked by the white square in the inset for position 6) are shown in Fig. 2 . Scale bars: 5 nm (main panel), 500 pm (inset). The rectangles at position 1, 2 and 6 indicate the areas of the topography maps in Fig. 4 and the inset. ( d ) Graphene edges. The two sublattices in the honeycomb structure are denoted A and B . The zigzag edge termination contains either A - or B -type atoms, whereas the armchair contains both types. ( e ) Atomic-resolution STM topography measured far from the edge shows the honeycomb structure with a slight intensity asymmetry on the two sublattices. Scale bar: 500 pm. ( f ) Intensity plot taken along the line in panel e displays an intensity modulation where one of the sublattices, marked A , appears 10% less intense than the other marked B . Full size image Graphene, a one-atom-thick crystal of carbon atoms arranged in a honeycomb lattice [25] , [26] , [27] , provides unprecedented opportunities to revisit the physics of QH edge states. The fact that its structure is strictly 2D, with electrons residing right at the surface, provides flexibility in choosing the distance to the screening plane. In typical devices, the graphene sample is deposited on a 300-nm-thick SiO 2 layer, capping a highly doped Si backgate [28] . In this configuration the confinement potential varies gradually over the screening length, l s , which is comparable to the thickness of the insulating spacer, leading to charge accumulation near the graphene edge over the same length scale [29] . When the spacer distance is much larger than the magnetic length ( ħ is the reduced Planck constant, −e is the electron charge and B is the magnetic field), as is the case in typical graphene devices, similar to the case in semiconductor-based 2DES, then the edge-state reconstruction is inevitable [29] . Here we show that edge-state reconstruction can be avoided when the graphene layer is very close to a screening plane. In this configuration the confining potential becomes atomically sharp. Thus, by controlling the thickness of the insulating spacer, it should be possible to carry out a systematic study of edge states under controlled screening conditions, which would allow testing theoretical ideas of QH edge physics [30] . Band structure and Landau levels in graphene The low-energy band structure of graphene, consisting of electron-hole symmetric Dirac cones, which touch at the Dirac points (DP) located at the K and K ′ corners (valleys) of the Brillouin zone, leads to a density of states (DOS), which is linear in energy and vanishes at the DP. In a magnetic field, B , normal to the graphene plane, the spectrum consists of a sequence of discrete Landau levels (LL): where N =0, ±1, ±2.. is the level index and is a characteristic energy scale. Here v F ~10 6 m/s is the Fermi velocity, ± refers to the electron/hole branches and E D is the energy of the DP measured relative to the Fermi energy. The LL spectrum in graphene is qualitatively different from that of the 2DES in semiconductors: it is electron-hole symmetric, displays square-root dependence on field and level index, and it contains an N =0 level, which reflects the chiral nature of the quasiparticles. The wave functions of the N =0 LL in valleys K and K ′ reside on different sublattices ( A or B ) of the honeycomb lattice. In finite size graphene samples, crystallographic edges can be either zigzag form, consisting of atoms belonging to only one sublattice, or armchair form that contains atoms from both ( Fig. 1d ). Samples and tunnelling spectra In this work we use low-temperature, high-magnetic field scanning tunnelling microscopy (STM) and spectroscopy (STS) to follow the spatial evolution of the local DOS in graphene supported on a graphite substrate [27] , [31] , [32] . As characterized previously [31] , the graphene flake is partially suspended over the graphite substrate at a distance ~0.44 nm, which is ~30% larger than that for AB (Bernal)-stacked graphite. This was found to suppress tunnelling between the layers so that the flake is electronically decoupled from the substrate and shows the hallmarks of intrinsic single-layer graphene: linear DOS that vanishes at the DP in zero field and an LL sequence with square-root dependence on magnetic field and level index [27] , [31] . The sample topography in Fig. 1c shows an edge, which is parallel to the zigzag direction as determined from the atomic-resolution image ( Fig. 1c inset). In the interior of the sample, the atomic-resolution image ( Fig. 1e ) reveals a well-resolved honeycomb structure. Plotted in Fig. 1f , the position dependence of the intensity along the dashed line indicated in Fig. 1e reveals an ~10% asymmetry between the two sublattices. LL spectra and their evolution towards a zigzag edge In the presence of a magnetic field, local LL spectra (averaged over an area 0.4 × 0.4 nm 2 ), shown in Fig. 2a , were taken starting from the edge and towards the bulk at the positions marked 1 to 6 in Fig. 1c , which were spaced by intervals of 6.5 nm=0.5 l B . Far from the edge, in the bulk of the sample, the spectra exhibit a series of pronounced peaks at energies that follow a square-root dependence on field and level index [31] , [33] as expected for the LL sequence of massless Dirac fermions (Equation (1)). In what follows, we discuss two notable features of the spectra: (a) the proximity of the edge is not felt up to a distance of ~2.5 l B , and then only as a subtle redistribution in spectral weight, whereas the peak positions remain unchanged; (b) the double peak corresponding to the split N =0 LL stands out in its robustness and persists all the way to the edge as expected for a zigzag termination. 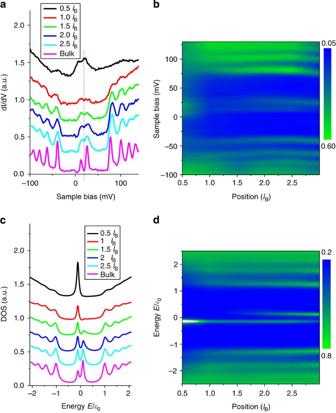Figure 2: Evolution of LLs with distance from the edge. (a) LL spectroscopy atB=4 T andT=4.4 K in the bulk and at the positions marked inFig. 1c. The energy origin is taken at the Fermi level. The dashed line indicates the bulk Dirac point energy. (b) LL maps showing the evolution of the spectra with distance from the edge. The colour scale encodes the magnitude of the measured differential conductance. (c) Simulated local DOS for the case ina, including broadening due to electron–electron interactions obtained in ref.31. (d) Simulated LL maps for the same parameters as in (b). Figure 2: Evolution of LLs with distance from the edge. ( a ) LL spectroscopy at B =4 T and T =4.4 K in the bulk and at the positions marked in Fig. 1c . The energy origin is taken at the Fermi level. The dashed line indicates the bulk Dirac point energy. ( b ) LL maps showing the evolution of the spectra with distance from the edge. The colour scale encodes the magnitude of the measured differential conductance. ( c ) Simulated local DOS for the case in a , including broadening due to electron–electron interactions obtained in ref. 31 . ( d ) Simulated LL maps for the same parameters as in ( b ). Full size image First, we consider the position of the peaks in the STS traces, which remain practically unchanged upon approaching the edge. This reflects the fact that the small screening length, determined by the distance to the graphite substrate ( l s ~0.4 nm), defines an essentially atomically sharp confinement potential. The connection between screening and the dispersion of the LL spectra with distance from the edge can be understood by considering the problem in the Landau gauge natural to the strip geometry. In this gauge, the high degeneracy of bulk LLs represents multiple choices for the position of the guiding centre, where L y is the width of the sample along the edge direction, y. For N =0 the electronic wavefunctions, , reside on only one sublattice, say A , whereas for higher-order indices, N ≠0, both sublattices carry the electronic wavefunctions that take the form on sublattice A, and on sublattice B . Here x , measured in units of l B , is the distance from the edge, and H N are the Hermite polynomials. The wavefunctions form strips of width that are centred on x m and run parallel to the edge. For guiding centres far from the edge, m »1, the states are identical to those in an infinite system. Near the edge, the wave functions are modified due to the boundary conditions and the degeneracy is lifted, [1] , [5] , [6] , [7] resulting in LLs bending away from the DP and the LL energy E Nm corresponding to ψ Nm now depends on the distance from the edge. This produces dispersive edge states, which, according to theory, carry the transport currents responsible for the QH effect [1] , [2] , [3] , [4] . The nature of the current-carrying states depends on the relative magnitudes of l s and l B . In the limit l s >> l B , accessed in the experiments on semiconductor-based 2DEG, the system lowers its energy by reconstructing the edge states into steps, as shown in Fig. 1a , which produce alternating compressible and incompressible strips [13] that carry the QH current and stabilize the QH plateaus even in the limit of a perfectly clean sample. Recent scanning probe microscopy experiments [20] , [21] , [22] , [23] have demonstrated the existence of these strips several magnetic lengths away from the edge. In the opposite limit, l s <<l B , the case of the experiments reported here, the strips are absent, and the N th LL shifts monotonically away from the DP for distances within of the edge [5] , [6] , [7] . For the case of a zigzag edge in graphene, there is one non-dispersive N =0 state confined to one of the valleys [6] . At larger distances from the edge x >> , the LL energies are identical to those in the bulk. The local DOS (LDOS) measured with STS is given by: where i is the sublattice index and r the position where the spectrum is taken. As the LDOS is determined not only by the energy but also by the wave functions, the edge spectrum is sensitive to the states in the bulk up to distances comparable to their spatial extent, x ~ . Because of the large degeneracy of the bulk states, they make an important contribution to the LDOS near the edge, so that the position of the peak in the LDOS is still very close to that in the bulk. Therefore, counter-intuitively, in this case the proximity to the edge appears not as a shift in the peak energy but as a redistribution of spectral weight from lower to higher energies. As a result, the amplitude of low-index peaks decreases faster than that of higher index peaks, even though the bending of high-index LLs is stronger (due to the greater spatial extent of the higher LL states). This hierarchical spectral weight redistribution, observed in both experimental and simulated data shown in Fig. 3 , is characteristic to bending of LLs near a sharp edge. Its presence makes it possible to distinguish experimentally between broadening due to edge disorder—which would affect all peaks equally—and level bending. 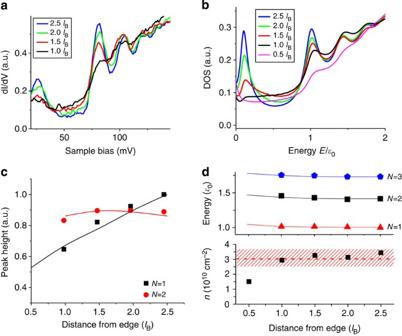Figure 3: Spectral weight redistribution near the sample edge. (a) Measured LL spectra atB=4 T showing the evolution of the peak heights with distance from the edge on the electron side at the positions marked inFig. 1c. (b) Simulated local DOS for the case in panela, including broadening due to electron–electron interactions obtained in ref.31. The local DOS is averaged over the two sublattices. Although the peaks corresponding to bulk LLs continue to dominate the local DOS down to 0.5lB, their amplitude decreases upon approaching the edge reflecting the spectral weight redistribution discussed in the text. (c) Spectral weight redistribution near the edge for both the experimental data (symbols) and the theory (solid lines) shows that the intensity of theN=1 peak decreases faster than that of theN=2 peak upon approaching the edge. (d) Top panel: comparison of measured evolution of LL peak positions with distance from the edge forN=1, 2, 3 (symbols) with calculated values (lines) for a sharp edge. Bottom panel: evolution of carrier density with distance from the edge shows no charge variation up to a distance of ~1lB. Figure 3: Spectral weight redistribution near the sample edge. ( a ) Measured LL spectra at B =4 T showing the evolution of the peak heights with distance from the edge on the electron side at the positions marked in Fig. 1c . ( b ) Simulated local DOS for the case in panel a , including broadening due to electron–electron interactions obtained in ref. 31 . The local DOS is averaged over the two sublattices. Although the peaks corresponding to bulk LLs continue to dominate the local DOS down to 0.5 l B , their amplitude decreases upon approaching the edge reflecting the spectral weight redistribution discussed in the text. ( c ) Spectral weight redistribution near the edge for both the experimental data (symbols) and the theory (solid lines) shows that the intensity of the N =1 peak decreases faster than that of the N =2 peak upon approaching the edge. ( d ) Top panel: comparison of measured evolution of LL peak positions with distance from the edge for N =1, 2, 3 (symbols) with calculated values (lines) for a sharp edge. Bottom panel: evolution of carrier density with distance from the edge shows no charge variation up to a distance of ~1 l B . Full size image Splitting of the N =0 LL Another notable feature of the data is the split N =0 peak and its persistence all the way to the edge, even while the others are smeared out. The splitting of the N =0 peak, most prominently seen in the bulk spectrum, was previously observed for graphene samples on graphite [27] , [31] , [32] , [33] and was attributed to a gap at the DP caused by substrate-induced breaking of the sublattice symmetry [27] . This broken symmetry is directly imaged in Fig. 1e as an intensity imbalance between the two sublattices. Its observation is consistent with the Bernal stacking between the monolayer graphene and the graphite substrate, which leads to a staggered potential on the A and B sublattices, and shifts the energies of the N =0 LL in the K and K ′ valleys in opposite directions. At first, it may seem surprising that the sublattice symmetry of the graphene layer can be broken by the substrate in spite of the absence of tunnelling between them. However, recalling that the broken symmetry is due to the electrostatic potential of the commensurate substrate, which decays much slower than the tunnelling probability, this scenario is consistent with the data. Theory For a quantitative comparison between theory and experiment, we simulate the spatial evolution of the LDOS close to a zigzag edge, including the level broadening due to the finite quasi-particle lifetime [31] . We use the low-energy continuum Dirac model [5] , [6] , [7] to obtain LL energies, wave functions and the LDOS by solving numerically two Dirac equations in magnetic field (one per each valley), supplemented by the boundary condition appropriate for the zigzag edge. In addition, we introduce splitting between N =0 Landau sublevels by imposing different potentials ±Δ on the two graphene sublattices. Furthermore, to account for the asymmetry of the split N =0 LL observed in the experiment, we assume that the tunnelling matrix element into the two sublattices is different. This could arise from the asymmetric coupling of two sublattices to the graphite substrate, consistent with the observed sublattice asymmetry observed in the topography maps. We found that taking p A =2 p B (here p A(B) is the squared matrix element for tunnelling into A ( B ) sublattice) gives the best agreement with experiment. Comparing with the measured LDOS in Figs 2 and 3 , we find that this simple model captures the main experimental features, including the evolution of the LL peak heights with distance from the edge ( Fig. 2c ) and the spectral weight redistribution ( Fig. 3b ). Consistent with the experimental data, the deviations from the bulk DOS appear only within ~2.5 l B of the edge as a redistribution of intensity without shifting the positions of the LL peaks. Another notable feature, also consistent with experiment, is the persistence of the strong double peak at the DP all the way to the edge, even while the others are smeared out. Tellingly, as the state at the DP persist in only one valley, the amplitude of one of the peaks in the N =0 doublet decreases for distances between 2.5 l B and 1 l B away from the edge. The local carrier density and sign can be obtained from the LL spectra by measuring the separation [25] between the Fermi energy ( E =0) and the DP ( E D ), which is identified with the centre of the two N =0 peaks. Far from the edge, the sample is hole doped, E D >0, with carrier density n ~3 × 10 10 cm −2 . From the position dependence of the LL spectrum and E D , we obtain in Fig. 3d the evolution of the local carrier density with distance from the edge. We note that the density remains practically unchanged upon approaching the edge to within ~1.0 l B , showing absence of edge reconstruction as expected for an edge with an atomically sharp confining potential. The agreement with this theory breaks down right on the edge, where the spectrum consists of three broad peaks seemingly unrelated to the bulk LLs ( Fig. 4a ). At the same time, atomic-resolution STM topography indicates a transition from honeycomb to triangular structure within ~ l B of the edge. We note the appearance, in the first few rows from the edge, of a stripe pattern that has the periodicity of the lattice consistent with the triangular structure seen further away ( Fig. 4c ). Similar striped structures were reported in STM topography measurements of graphite edges [34] . The spectroscopic and topographic features reported here are qualitatively similar to zero-field density-functional calculations of the charge distribution near a pure zigzag edge of graphene [35] . Both exhibit a transition from a triangular structure with a stripe-like pattern near the edge to a honeycomb structure further away. Remarkably, the calculation reveals the presence of three low-energy flat bands, which produce three peaks in the edge DOS similar to the ones observed here. The highest energy peak is produced by the flat band that emerges from the bulk π electrons and is localized at the edge, whereas the two lower-energy peaks arise from the dangling bonds. Although these simulations exhibit a striking overall similarity to the data, the predicted energy of the peaks exceeds the measured energy by about a factor of two. To address this discrepancy, future work would require taking into account an edge that is not perfectly zigzag, the graphite substrate, the possibility of adsorbed atoms and the presence of the magnetic field. 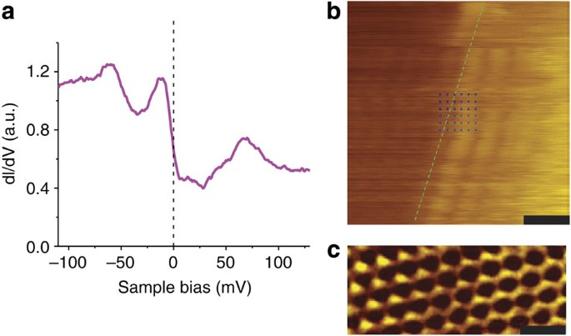Figure 4: STM/STS at a zigzag edge. (a) Differential conductance spectrum on the edge is singularly different from the spectra inside the sample shown inFig. 2. The spectrum was averaged over locations marked by the dots in panelb. (b) Topography at the zigzag edge (position 1 inFig. 1cmarked by red square). (c) Zoom-in near position 2 marked by red rectangle inFig. 1c(~6.5 nm away from the edge) shows a transition from a honeycomb to triangular structure. Scale bars: 500 pm inbandc. Figure 4: STM/STS at a zigzag edge. ( a ) Differential conductance spectrum on the edge is singularly different from the spectra inside the sample shown in Fig. 2 . The spectrum was averaged over locations marked by the dots in panel b . ( b ) Topography at the zigzag edge (position 1 in Fig. 1c marked by red square). ( c ) Zoom-in near position 2 marked by red rectangle in Fig. 1c (~6.5 nm away from the edge) shows a transition from a honeycomb to triangular structure. Scale bars: 500 pm in b and c . Full size image In summary, this work shows that when the screening plane is very close to 2DES as in the case of graphene on graphite, the QH edge states display the characteristics of confinement by an atomically sharp edge. The absence of edge-state reconstruction demonstrated here indicates that graphene is a suitable system for realizing one-dimensional chiral Luttinger liquid states and for probing their universal properties as a projection of the underlying QH state. The findings reported here, together with the techniques available to control the local density and the screening geometry in graphene, guarantee that edge softness and its undesirable reconstruction could be overcome in future experiments by using a combination of gating across a tunable gap in suspended samples and side gates [36] , or by using a thin boron nitride crystal as a spacer between graphene and the backgate [37] . This new type of unreconstructed edge states will provide a test-bed for the theoretical ideas and can open new avenues for exploring the physics of the one-dimensional QH channels. Sample preparation and characterization STM tips were mechanically cut from Pt-Ir wire. The tunnelling conductance dI/dV was measured using lock-in detection at 340 Hz. A magnetic field, 4 T, was applied perpendicular to the sample surface. Typical tunnelling junctions were set with 300 mV sample bias voltage and 20 pA tunnelling current. The samples were obtained from highly oriented pyrolitic graphite cleaved in air and immediately transferred to the STM. In addition to removing surface contamination, this methods often leave graphene flakes on the graphite surface, which are decoupled or weakly coupled to the substrate. The graphene flakes are characterized with topography followed by finite-field spectroscopy in search of a well-defined and pronounced single sequence of LLs, indicating decoupling from the substrate [31] . Coupling between layers, even when very weak, gives rise to additional peaks whose position reflects the degree of coupling [27] , [31] , [32] . How to cite this article: Li, G. et al . Evolution of Landau levels into edge states in graphene. Nat. Commun. 4:1744 doi: 10.1038/ncomms2767 (2013).